Conformational fitting of a flexible oligomeric substrate does not explain the enzymatic PET degradation 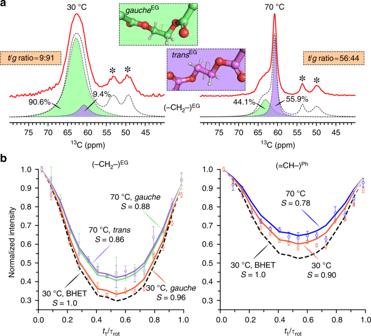Fig. 1 MAS NMR of amorphous PET powder at 30 °C and 70 °C.a13C spectra in the range of 40–80 ppm showing the characteristic spectra for the EG carbons. Thetransandgauchecontents were quantified by fitting a Voigt function to the experimental spectra (red). The sum of the Voigt fits (shaded in purple and green, respectively, fortransandgaucheconformers) is shown as dotted curve. The inset shows the EG fragment in thetransandgaucheconformations. MAS sidebands are denoted by asterisks.b1H–13C DIPSHIFT curves for phenylene and EG carbons acquired at a MAS rate of 8 kHz. The solid lines are the best-fit simulations and dashed lines represent the rigid limit. Experimental error bars were determined from the noise level. Order parametersSfrom the measured dipolar couplings are given. 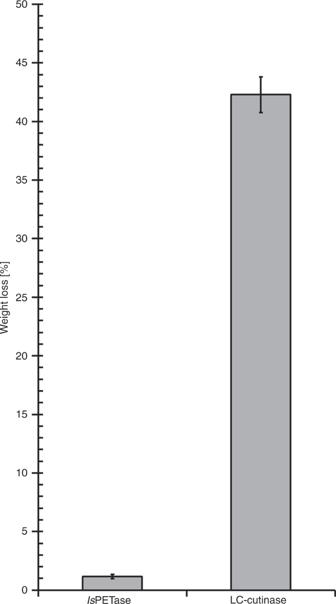Fig. 2 Weight loss of an amorphous PET film (~45 mg) as a result of enzymatic hydrolysis. Incubation withIsPETase and LC-cutinase was carried out under agitation for 24 h at 30 °C and 70 °C, respectively, i.e., at their optimal reaction conditions for PET degradation. Error bars indicate the standard deviation of triplet measurements. Solid-state NMR analysis of amorphous PET powder Amorphous PET films (product no. ES301445) were purchased from Goodfellow Cambridge Ltd. (Huntingdon, UK) and ground in a cryomill in the presence of liquid nitrogen. Particles with diameters of less than 0.25 mm were obtained by sieving and then used in the solid-state NMR analysis. All CP/MAS (cross-polarization magic-angle spinning) NMR experiments were performed at 9.4 T with a Bruker AVANCE III NMR spectrometer equipped with a 4-mm double-resonance MAS probe (Rheinstetten, Germany). A MAS rate of 8 kHz was maintained throughout the experiments. The 207 Pb NMR resonance of lead nitrate was used as the thermometer to calibrate the temperature over the sample volume of the in-situ MAS probe at 8 kHz [12] . The MAS data were acquired respectively at 30 and 70 °C by using two individual samples. Each fine-powdered PET sample (~30 mg) was loaded into a 4 mm ZrO 2 MAS rotor with Vespel cap and incubated at their individual target temperatures in the magnet for 24 h prior to the data acquisition. Optimized 1 H and 13 C 90° pulse lengths were 2.5 and 3.0 μs, respectively. The CP/MAS spectra were recorded with 2512 scans and a relaxation delay of 4 s, with optimized spin-lock pulses to satisfy both Hartmann–Hahn (HH) n = ±1 matching conditions, with 66 kHz effective 13 C radio frequency (r.f.) lock field and 100–70% ramp on the 1 H channel. Decomposition of methylene carbon resonances from the EG units provided direct quantification for the t / g ratio. The contact time was 2 ms. 1 H– 13 C order parameters were measured using the 2D DIPSHIFT experiments [5] . The experiments were conducted with 256 scans and a recycle delay of 4 s. 1 H– 1 H homonuclear dipolar decoupling was accomplished with phase-modulated Lee–Goldburg (PMLG) approach [13] . The PMLG block consists of 10 pulses with the following phases: 339.22°, 297.65°, 256.08°, 214.51°, 172.94°, 352.94°, 34.51°, 76.08°, 117.65°, and 159.22° (m5m shape in TopSpin library, Bruker). The PMLG5-optimized pulse was 2.07 μs and the r.f. decoupling field was set to 80 kHz. The PMLG scaling factor of 0.5 was determined based on adamantane J -splitting. For all experiments, swept-frequency two-pulse phase-modulation (SW f -TPPM) heteronuclear decoupling [14] with a r.f. field of 100 kHz was used during the acquisition. 13 C chemical shifts were externally referenced to the C(=O)O − signal of solid tyrosine·HCl at 172.1 ppm. The DIPSHIFT dephasing curves were simulated using the SIMPSON program [15] . The rigid-limit values for both CH and CH 2 spin systems were obtained by fitting the experimental curves of crystalline BHET in a site-specific manner. Spectral fitting was conducted with the MestReNova 12.0.0 program (Mestrelab Research, Santiago de Compostela, Spain). Enzymatic hydrolysis of amorphous PET films A codon-optimized synthetic gene encoding Is PETase lacking the N-terminal signal sequence containing 27 residues was ordered from Genscript (Piscataway, USA) and subcloned into the pET-21b vector (Novagen, San Diego, USA). The recombinant Is PETase containing a C-terminal His 6 -tag was expressed in Escherichia coli Shuffle T7 Express (New England Biolabs GmbH, Frankfurt am Main, Germany). Briefly, E. coli cells were grown at 30 °C to an optical density (OD 600 ) of 1, followed by induction in the presence of 0.1 mM IPTG at 16 °C for more than 12 h, and then purified by immobilized metal ion chromatography (IMAC) using TALON metal affinity resin (Takara Bio Europe, Saint-Germain-en-Laye, France) to homogeneity. LC-cutinase was recombinantly expressed in E. coli BL21(DE3) and purified by IMAC to homogeneity using Ni-NTA (Qiagen, Hilden, Germany) as previously described [16] . 5 μg of Is PETase and 50 µg of LC-cutinase were used to degrade a piece of amorphous PET film (Goodfellow Cambridge Ltd., 3 × 0.5 cm 2 , ~45 mg) using the optimal degradation conditions for the respective enzymes [2] , [16] . Briefly, Is PETase required 50 mM Na 2 HPO 4 -HCl at pH = 7 while LC-cutinase required 1 M K 2 HPO 4 /KH 2 PO 4 at pH = 8. Degradation was performed by shaking the reaction vials on a thermoshaker TS1 (Biometra, Göttingen, Germany) at 1000 rpm for 24 h at 30 °C for Is PETase and at 70 °C for LC-cutinase. The reaction was stopped by cooling the samples on ice. PET films were washed sequentially with 0.1% aqueous SDS, ethanol and ultrapure water and then dried at 50 °C for 48 h before subjected to gravimetric weight loss determination. Degradation experiments using higher Is PETase concentrations up to 50 µg enzyme and lower LC-cutinase amount down to 5 µg enzyme were also prepared as control samples which led to significantly lower weight losses of the PET films (data not shown) than using the enzyme amounts mentioned above in main text.